Epigenetic variation in theEgfrgene generates quantitative variation in a complex trait in ants Complex quantitative traits, like size and behaviour, are a pervasive feature of natural populations. Quantitative trait variation is the product of both genetic and environmental factors, yet little is known about the mechanisms through which their interaction generates this variation. Epigenetic processes, such as DNA methylation, can mediate gene-by-environment interactions during development to generate discrete phenotypic variation. We therefore investigated the developmental role of DNA methylation in generating continuous size variation of workers in an ant colony, a key trait associated with division of labour. Here we show that, in the carpenter ant Camponotus floridanus , global (genome-wide) DNA methylation indirectly regulates quantitative methylation of the conserved cell-signalling gene Epidermal growth factor receptor to generate continuous size variation of workers. DNA methylation can therefore generate quantitative variation in a complex trait by quantitatively regulating the transcription of a gene. This mechanism, alongside genetic variation, may determine the phenotypic possibilities of loci for generating quantitative trait variation in natural populations. Understanding how variation in quantitative traits is generated is important for mapping the genetic basis of disease, improving plant and animal breeding, and predicting evolutionary changes [1] , [2] . The field of quantitative genetics has produced a wealth of knowledge regarding the genetic basis of quantitative trait variation, including the number, distribution and identification of large and small effect loci underlying quantitative traits [1] , [2] , [3] . Little is known, however, about how the environment interacts with such loci and whether this interaction can generate quantitative trait variation [4] , [5] . Several studies have shown that epigenetic mechanisms, such as DNA methylation and histone modifications, can mediate gene-by-environment interactions during development to generate discrete phenotypic variation [6] , [7] , [8] , [9] . For example, in rats, DNA methylation mediates the onset of stress tolerance in response to the presence/absence of postnatal maternal care [8] , and in social insects, DNA methylation plays a role in regulating discrete morphological [7] and behavioural [10] differences between queen and worker castes. It remains unclear, however, what role DNA methylation plays in generating quantitative trait variation. Here, we use ant societies to address this question because continuous variation in the size of individuals in the worker caste is a key trait associated with the division of labour, where differently sized workers can specialize in tasks such as excavation, brood transport and foraging [11] , [12] , [13] . All holometabolous insects (ants, bees, wasps, beetles, butterflies, moths and flies) do not grow as adults [14] , [15] . All growth occurs during the larval phase when larvae molt from one instar to the next and during each instar [14] , [15] . Adults, due to their tough inflexible exoskeleton, do not molt and therefore their final body size is determined entirely by the end of larval development just before metamorphosis [14] , [15] . The final size of a worker in an ant colony is therefore established during development [16] . Determination of final size of a worker is polyphenic, which means that the same genome can produce a spectrum of final adult sizes in response to environmental factors [11] , [16] , [17] . Studies in the wild and in the lab spanning more than 100 years have identified nutrition levels and social interactions as critical environmental factors that influence the final size of workers during larval development [16] , [17] , [18] , [19] . In ant species where genetic variation in the worker caste has been shown to be high, worker larvae in the colony remain polyphenic, but may vary quantitatively in their response to these environmental factors [20] , [21] , [22] . In the ant genus Camponotu s, variation in worker size has been shown to be influenced by nutrition in the form of protein, vitamins and minerals [23] , [24] . We chose the ant species C. floridanus because worker size variation is continuous, genetic variation between workers in a C. floridanus colony is low (workers are on average 75% related) [25] and extensive sequencing efforts indicate that within a colony there is no allelic bias between differently sized workers [26] . Therefore, genetic variation alone cannot fully explain the diversity of worker size found in C. floridanus . Finally, the genome of C. floridanus is sequenced and has a DNA methylation system [26] , [27] , thereby making this species an excellent model for understanding how gene-by-environment interactions generate quantitative trait variation in natural populations. DNA methylation in vertebrates occurs in regulatory elements that reside in promoter regions as well as inside and outside of gene bodies throughout the genome [28] , [29] , and is known to repress gene function through the covalent modification of cytosine residues within these elements [30] . In social insects, however, DNA methylation occurs primarily in gene bodies [28] , [29] , [31] and is generally associated with caste-specific alternative splicing [26] , [32] , [33] and gene expression [7] , [32] . There is functional evidence in honeybees that gene body methylation regulates alternative splicing [34] and can repress gene expression and phenotype [7] in a caste-specific manner. Knockdown of a DNA methylating enzyme ( Dnmt3 ) in adult honeybee fat tissue affects alternative splicing [34] , whereas knockdown of this enzyme in developing honeybee larvae results in the appearance of queen-like morphologies and a change in transcription levels of several types of genes, including those involved in growth and metabolism [7] . One of these growth-regulating genes Target of rapamycin ( Tor ) is more methylated [33] and is expressed at lower levels [35] in developing workers than in queens. Knockdown of tor in queen-destined larvae results in adults with worker characteristics [35] , indicating that gene body methylation is involved in repressing the expression of Tor in workers. In this study, we examine the hypothesis that naturally occurring inter-individual differences in a quantitative trait can also be generated by environmental variation through quantitative inter-individual differences in DNA methylation. We show that in colonies of the ant C. floridanus , natural inter-individual variation in the size of workers correlates with the natural inter-individual variation in the state of methylation of the highly conserved gene Egfr . We performed functional experiments to demonstrate that genome-wide DNA methylation indirectly regulates the quantitative methylation of Egfr to generate quantitative variation in the size of workers. By linking a continuous distribution in a trait in a natural population with a continuous distribution of DNA methylation states in a single gene, our study provides an epigenetic mechanism for generating quantitative variation in organismal phenotypes. Worker size variation and development in natural populations To address the role that DNA methylation plays in the regulation of worker size variation in C. floridanus , we first determined the size distribution of adult workers. We found that it is continuous with two peaks in frequency that represent the two worker subcastes—minor ‘m’ and major ‘M’ workers [11] in Fig. 1a,b . Although all workers form a continuous size distribution, minors and majors are distinguished by head allometry (the size of their heads relative to their bodies; Fig. 1c ). To identify the developmental stage where this dramatic variation in worker size is established, we determined the number of larval instars. We found that there are a total of four larval instars and that most of the growth differences in size between workers are established during the 4th (final) instar ( Fig. 1d ). The early 4th instar larvae have not yet experienced this rapid growth (‘early’ in Fig. 1d ), whereas late 4th instar larvae undergo a burst of growth producing a continuous range of final larval sizes ( Fig. 1d ). Because final adult size is determined at the end of larval development in insects [14] , [15] , including ants [16] , we can therefore infer that the smaller larvae (‘m’ in Fig. 1d ) will develop into adult minor workers, whereas the larger larvae (‘M’ in Fig. 1d ) will develop into major workers. 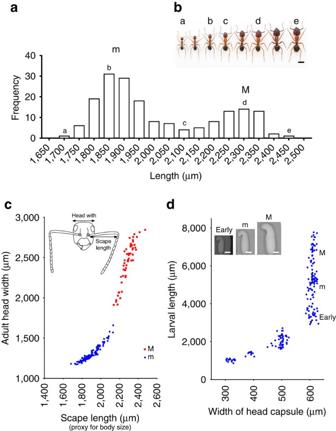Figure 1: Continuous size distribution of workers inC. floridanus. (a) Continuous distribution of adult size ofC. floridanusworkers (n=179). This distribution is based on scape length (b), a common proxy for body size. (b) Representative categories of sizing continuum in naturalC. floridanuspopulations that exists from smallest a to largest e. Magnification is × 8. (c) Allometric classification of adultC. floridanusworkers into major and minor workers. Adult head width was plotted against adult scape length. Minor and major adult workers are distinguished by a break in the allometry curve. Blue circles indicate minor workers, red squares indicate major workers. (d) Developmental stages and establishment of final worker sizes (n=197); minor worker-destined larvae are indicated by m and major worker-destined larvae are indicated by M. Magnification of inset is × 30. Figure 1: Continuous size distribution of workers in C. floridanus . ( a ) Continuous distribution of adult size of C. floridanus workers ( n =179). This distribution is based on scape length ( b ), a common proxy for body size. ( b ) Representative categories of sizing continuum in natural C. floridanus populations that exists from smallest a to largest e. Magnification is × 8. ( c ) Allometric classification of adult C. floridanus workers into major and minor workers. Adult head width was plotted against adult scape length. Minor and major adult workers are distinguished by a break in the allometry curve. Blue circles indicate minor workers, red squares indicate major workers. ( d ) Developmental stages and establishment of final worker sizes ( n =197); minor worker-destined larvae are indicated by m and major worker-destined larvae are indicated by M. Magnification of inset is × 30. Full size image Worker size variation is linked to DNA methylation We then tested if differential methylation at the genomic and gene levels during development may be involved in generating the continuous distribution of worker size in C. floridanus . Before examining the entire size continuum, however, we first used the extreme ends of the distribution to screen for dynamic changes in global DNA methylation that are associated with the early and late phases of larval growth during the 4th instar. If DNA methylation plays a role in regulating worker size variation, then we expected to find higher levels of methylation in the smallest worker larvae and lower levels of methylation in the largest worker larvae. Indeed, we found that early 4th instar larvae have significantly lower levels of global methylation relative to late 4th instar larvae ( Fig. 2a ) and 4th instar minor worker larvae were significantly hypermethylated compared with 4th instar major worker larvae ( Fig. 2a ). We next compared expression levels of key enzymatic regulators of DNA methylation [9] (DNA methyltransferase 1 ( Dnmt1 ), DNA methyltransferase 3 ( Dnmt3 ), Ten-eleven-translocation 2 ( Tet2 ), Methyl-binding domain ( Mbd ) and Methyl CpG-binding protein 2 ( Mecp2 )) and histone modification [9] (Histone deacetylase 1 ( Hdac1 ), Histone deacetylase 3 ( Hdac3) , Histone acetyltransferase ( Hat ) and Lysine-specific demethylase 1 ( Lsd1 )) and asked whether alterations in the level of expression of these regulators correspond to differences in global DNA methylation. We found that differences in levels of gene expression of Dnmt1 , Dnmt3 , Tet2 , Mbd and Mecp2 ( Fig. 2b,c and Supplementary Fig. 1a–d ) as well as Hdac1 and Hat ( Supplementary Fig. 1d,f ) correspond to differences in global methylation levels during the 4th instar. Considering that key enzymatic regulators of DNA methylation, Mbd and Mecp2 , are known to interact with HDACs [36] , both regulators of DNA methylation and histone modification may contribute to the pattern of global DNA methylation. Our results therefore suggest a link between global DNA methylation and the regulation of the continuous worker size variation during the fourth instar in C. floridanus . 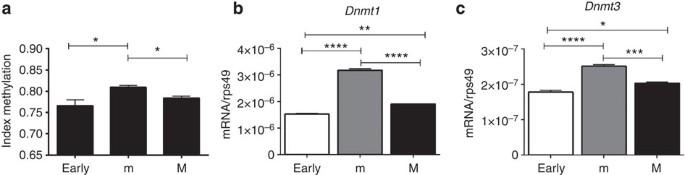Figure 2: DNA methylation profiles during development. (a) Genomic methylation in early 4th instar, as well as minor and major larvae in late 4th instar. Genomic methylation is shown as a ratio of [MspI/HpaII] cuts to provide an index of overall DNA methylation. Transcription level of (b)Dnmt1and (c)Dnmt3in early 4th instar larvae (white bar), late minor worker larvae (grey bar) and late major worker larvae (black bar). Bars indicate mean, whereas error bars indicate±s.e.m. Statistical significance values for Student’st-test are as follows: *P<0.05, **P<0.01, ***P<0.001, ****P<0.0001. Sample sizes for each larval category isn≥30 individual larvae. Figure 2: DNA methylation profiles during development. ( a ) Genomic methylation in early 4th instar, as well as minor and major larvae in late 4th instar. Genomic methylation is shown as a ratio of [MspI/HpaII] cuts to provide an index of overall DNA methylation. Transcription level of ( b ) Dnmt1 and ( c ) Dnmt3 in early 4th instar larvae (white bar), late minor worker larvae (grey bar) and late major worker larvae (black bar). Bars indicate mean, whereas error bars indicate±s.e.m. Statistical significance values for Student’s t -test are as follows: * P <0.05, ** P <0.01, *** P <0.001, **** P <0.0001. Sample sizes for each larval category is n ≥30 individual larvae. Full size image DNA methylation regulates worker size variation To determine whether global DNA methylation plays a functional role during development to regulate the continuous size variation of workers, we manipulated levels of global methylation during the early 4th instar. We used a hypomethylating agent, the inhibitor of DNA methyltransferases 5-AZA-dCytidine (5-AZA-dC) [37] , and a hypermethylating agent, the methyl donor S -adenosyl methionine [38] (SAM). Relative to controls, we found that 5-AZA-dC significantly reduced genomic methylation ( Supplementary Fig. 3a ) and shifted the continuous size distribution by significantly increasing the mean size of adult workers ( Fig. 3b,e,f , Supplementary Fig. 2a–c ). In contrast, we found that SAM increased genomic methylation as expected (although not statistically significant; Supplementary Fig. 3b ) and shifts the continuous size distribution by significantly decreasing the mean size of adult workers ( Fig. 3a,c,d and Supplementary Fig. 2d–f ). Although SAM has many biological functions, its role in mediating global DNA methylation and sizing is reinforced by the contrasting effect on genomic methylation levels and phenotype caused by 5-AZA-dC, a well-known hypomethylating agent. Finally, because worker size is sensitive to environmental conditions (nutrition and social interactions), the size range of workers emerging from our control replicates is always smaller than in our lab-reared wild-type colonies (see insets Fig. 3a,b ). This means that we are generally underestimating the magnitude of the effect of these drug treatments on shifting the continuous size distribution of workers ( Figs 1a and 3a,b ). These results demonstrate that, during larval development, global DNA methylation is involved in regulating continuous worker size distribution in C. floridanus . 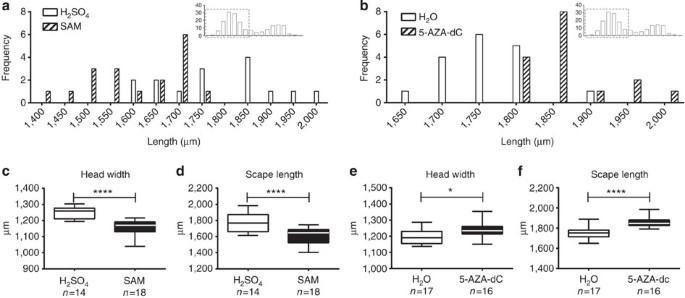Figure 3: Pharmacological manipulation of global (genome-wide) DNA methylation shifts mean of continuous worker size distribution. Hatched bars indicate effect of (a) SAM (n=18) and (b) 5-AZA-dC (n=16) administration at the early 4th instar, whereas white bars indicate controls (H2SO4for SAM and H2O for 5-AZA-dC) relative to WT distribution of sizes seen in inset. SAM-treated animals (black box) compared with control (white box;n=14) for (c) head width and (d) scape length. 5-AZA-dC-treated (black box) animals compared with control (white box;n=17) for (e) head width and (f) scape length. Boxplot whiskers indicate min and max. Box defined by 25th percentile, mode and 75th percentile. Bars indicate mean and error bars indicate±s.e.m. Statistical significance values for Student’st-test are as follows: *P<0.05, ****P<0.0001. Note that all scape length and head width measurement data are normally distributed (tested with Shapiro-Wilk’s test). Figure 3: Pharmacological manipulation of global (genome-wide) DNA methylation shifts mean of continuous worker size distribution. Hatched bars indicate effect of ( a ) SAM ( n =18) and ( b ) 5-AZA-dC ( n =16) administration at the early 4th instar, whereas white bars indicate controls (H 2 SO 4 for SAM and H 2 O for 5-AZA-dC) relative to WT distribution of sizes seen in inset. SAM-treated animals (black box) compared with control (white box; n =14) for ( c ) head width and ( d ) scape length. 5-AZA-dC-treated (black box) animals compared with control (white box; n =17) for ( e ) head width and ( f ) scape length. Boxplot whiskers indicate min and max. Box defined by 25th percentile, mode and 75th percentile. Bars indicate mean and error bars indicate±s.e.m. Statistical significance values for Student’s t -test are as follows: * P <0.05, **** P <0.0001. Note that all scape length and head width measurement data are normally distributed (tested with Shapiro-Wilk’s test). Full size image EGFR regulates worker size variation To identify potential targets of DNA methylation, we assayed the expression of a panel of genes (Juvenile hormone acid methyltransferase ( JHAMT2 ), Juvenile hormone esterase ( JHE2 ), Target of rapamycin ( Tor ), Phosphatase and tensin homologue ( Pten ), chico , Epidermal growth factor receptor ( Egfr )) from pathways known to play critical roles in regulating discrete size differences in social insects ( Supplementary Fig. 4 ) [35] , [39] , [40] , [41] . We found that Egfr shows the most dramatic increase in expression within 4th instar minor worker larvae ( Fig. 4a and Supplementary Fig. 4f ). EGFR acts as a cell surface receptor that binds specific extracellular protein ligands, including growth factors from the epidermal growth factor and transforming growth factor (alpha) families. Once bound, EGFR stimulates phosphorylation and activates downstream pathways, including the Mitogen-activated protein kinase, Serine-threonine protein kinase and c-Jun N-terminal kinase pathways, leading to the regulation of DNA synthesis, growth, cell proliferation, differentiation and many other vital cellular processes [42] . In honeybees, dietary cues (royal jelly) stimulate EGFR signalling, which regulates size and developmental timing, leading to the development of queens [39] . Furthermore, in fruit flies, mapping loci that underlie quantitative traits (quantitative trait loci or QTLs) has identified Egfr as a genetic locus with a major effect on variation in quantitative sizing [43] . To determine the developmental role of EGFR in regulating the continuous variation in worker size in C. floridanus , we inhibited EGFR signalling during the early 4th instar using a pharmacological inhibitor (PD 153035). This inhibitor is known to be specific to EGFR [44] , and as expected, significantly inhibits EGFR phosphorylation 24 h post treatment ( Supplementary Fig. 3c,d ). We discovered that, relative to controls, inhibition of EGFR shifts the continuous size distribution by significantly increasing the mean size of adult workers ( Fig. 4c–e and Supplementary Fig. 2g–i ). This dramatic effect of EGFR inhibition indicates that EGFR is involved in regulating the continuous size distribution of workers in C. floridanus . 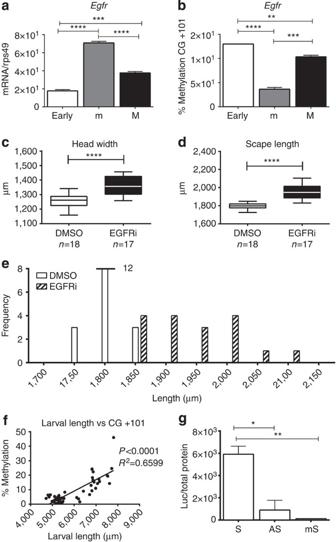Figure 4: The role and regulation ofEgfrin generating quantitative variation in worker size. (a)Egfrexpression in early 4th (white bar), late 4th instar minor (grey bar) and major larvae (black bar;n≥30). (b) Percent (%) methylation of site CpG +101 inEgfrfor early 4th instar (white bar), late 4th instar minor (grey bar) and major larvae (black bar;n≥30). EGFR inhibition of early 4th instar worker larvae (black box) compared with control DMSO (white box) for (c) head width and (d) scape length. Scape and head width measurement data are normally distributed (tested with Shapiro-Wilk’s test). Boxplot whiskers indicate min and max. Box defined by 25th percentile, mode and 75th percentile. (e) EGFR inhibition at the early 4th instar and its effect on sizing distribution (hatched bars;n=17) compared with control DMSO (white bars;n=18) relative to WT distribution of sizes seen in inset. (f) Linear regression between percent (%) methylation ofEgfrsite +101 (y-axis) and final larval length in μm (x-axis) across a spectrum of larval sizes (n=50). (g)Egfrpromoter cloned into luciferase reporter pCpGl in sense (S), antisense (AS) and methylated sense (mS). Bars indicate luciferase activity from the pCpGl construct relative to total protein (n=3). Data shown as mean and error bars indicate±s.e.m. Statistical significance values for Student’st-test are as follows: *P<0.05, **P<0.01, ***P<0.001, ****P<0.0001. Figure 4: The role and regulation of Egfr in generating quantitative variation in worker size. ( a ) Egfr expression in early 4th (white bar), late 4th instar minor (grey bar) and major larvae (black bar; n ≥30). ( b ) Percent (%) methylation of site CpG +101 in Egfr for early 4th instar (white bar), late 4th instar minor (grey bar) and major larvae (black bar; n ≥30). EGFR inhibition of early 4th instar worker larvae (black box) compared with control DMSO (white box) for ( c ) head width and ( d ) scape length. Scape and head width measurement data are normally distributed (tested with Shapiro-Wilk’s test). Boxplot whiskers indicate min and max. Box defined by 25th percentile, mode and 75th percentile. ( e ) EGFR inhibition at the early 4th instar and its effect on sizing distribution (hatched bars; n =17) compared with control DMSO (white bars; n =18) relative to WT distribution of sizes seen in inset. ( f ) Linear regression between percent (%) methylation of Egfr site +101 ( y -axis) and final larval length in μm ( x -axis) across a spectrum of larval sizes ( n =50). ( g ) Egfr promoter cloned into luciferase reporter pCpGl in sense (S), antisense (AS) and methylated sense (mS). Bars indicate luciferase activity from the pCpGl construct relative to total protein ( n =3). Data shown as mean and error bars indicate±s.e.m. Statistical significance values for Student’s t -test are as follows: * P <0.05, ** P <0.01, *** P <0.001, **** P <0.0001. Full size image DNA methylation regulates worker size variation through EGFR To determine whether global DNA methylation developmentally regulates continuous size distribution in workers through EGFR, we assayed Egfr methylation and expression levels after we experimentally treated early 4th instar larvae with SAM and 5-AZA-dC. We found an inverse relationship between levels of global DNA methylation and Egfr expression. Increasing global methylation by SAM treatment during the 4th larval instar results in decreased methylation and increased expression of Egfr ( Supplementary Fig. 5a,b ), whereas decreasing global methylation by 5-AZA-dC treatment results in increased methylation and decreased expression of Egfr ( Supplementary Fig. 5c,d ). This indicates that other intermediate genes or processes downstream to global changes in DNA methylation state mediate this inverse relationship [45] , [46] . Furthermore, DNA methylation and EGFR signalling may regulate worker size differences by affecting developmental timing. In ants, increasing the duration of development gives worker larvae more time to grow resulting in larger adult workers, whereas decreasing the duration of development gives larvae less time to grow resulting in smaller adult workers [47] . We found that the duration of development was shortened following SAM treatment, whereas it was extended after EGFR inhibition ( Supplementary Fig. 6a,c ). 5-AZA-dC did not affect developmental timing possibly because higher concentration may be required to elicit such a response or because 5-AZA-dC affects on sizing may operate through a developmental timing-independent mechanism. Our results indicate that global DNA methylation indirectly regulates the expression and methylation levels of Egfr during development, which in turn regulates the continuous size distribution of workers possibly through changes in developmental timing. Quantitative methylation of Egfr generates worker size variation We then discovered that DNA methylation through the specific methylation of Egfr not only regulates, but also generates a large part of the continuous worker size distribution. We found that quantitative differences in DNA methylation of Egfr is highly correlated to the final size of individual worker larvae, which spans the entire larval size range of the distribution, including minor and major worker larvae. Because final adult size is determined at the end of larval development [14] , [15] , [16] , we can therefore infer that these quantitative differences in DNA methylation of Egfr are also correlated to final adult size. In the C. floridanus genome, CpG dinucleotide methylation is primarily concentrated at the beginning of the protein-coding region of all genes [26] . We therefore screened the first 225 bp of Egfr and identified all CpG dinucleotides. We then determined the % methylation for each of these CpG dinucleotides in 50 individual late 4th instar larvae that represent the entire size continuum of workers. Of all the CpG dinucleotides screened, we discovered four sites for which the level of DNA methylation is significantly correlated to the final size of late 4th instar larvae ( Fig. 4b,f and Supplementary Fig. 7 ). Two of these sites (CG +101, R 2 =0.66 and CG +182, R 2 =0.24) remained statistically significant after Bonferroni correction for multiple comparisons ( Supplementary Fig. 7 and Supplementary Table 2 ). We then cloned this sequence into a CpG-free luciferase construct to determine whether these CpG dinucleotides, when methylated, affect the transcription of Egfr . We show that this differentially methylated region of Egfr could direct the transcription of this luciferase reporter in human HEK293 cells suggesting that it is a bona fide transcription regulatory region and that DNA methylation can indeed repress its transcriptional activity ( Fig. 4g ). Finally, in order to rule out sequence variation in this region of Egfr as a possible cause for the observed size differences of individual workers, we sequenced this region from the smallest (minor) and the largest (major) workers and found no genetic differences ( Supplementary Fig. 8 ). Collectively, our results indicate that DNA methylation quantitatively regulates Egfr during larval development to generate a large part of the continuous worker size distribution. Generation of continuous worker size variation by the epigenetic control of Egfr can be hypothesized as follows ( Fig. 5 ): variation in environmental factors leads to the hypermethylation (increase) or hypomethylation (decrease) of genomic DNA methylation levels during development of final instar larvae. Although our study did not determine the specific environmental factors that cause natural variation in DNA methylation, previous studies in ants, including other species in the genus Camponotus , have established both nutritional variation and social interactions as causes for variations in worker size [16] , [17] , [18] , [19] , [23] , [24] . Hyper- or Hypo-methylation in genomic DNA methylation levels then translates into the differential quantitative methylation of Egfr through intermediary genes or processes. Histone modifications are known to be key regulators in C. floridanus [48] , making them a possible candidate for this intermediary regulation of the inverse relationship between global DNA methylation and methylation of Egfr . This results in quantitative inter-individual differences in the transcription of Egfr in the colony, which in turn generates the differential growth attained by late final instar larvae. In C. floridanus , we show that quantitative methylation at Egfr explains a large proportion of the variance (>65%) of final larval size in natural colonies. This, combined with our drug treatment results and the fact that final adult size is determined by the final size of larvae [14] , [15] , suggests a causal relationship between methylation, Egfr , and the final size of adult workers. 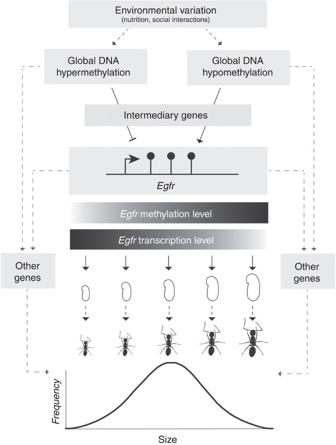Figure 5: Model for the generation of a continuous distribution of worker size through quantitative DNA methylation ofEgfr. Solid black lines indicate our results, whereas dashed black lines indicate our inferences from the literature. Lines with perpendicular tips indicate repression, whereas lines with arrowheads indicate activation. Environmental variation may lead to either global DNA hyper- or hypo-methylation (dashed black lines). Intermediary genes or processes quantitatively modulate this global DNA methylation state (solid black lines) into a specific level ofEgfrmethylation (black lollipops and box with increasing gradient from left to right, where an increase in black corresponds to increasing levels of methylation), which results in a specific level ofEgfrtranscription level (box with decreasing gradient from left to right, where a decrease in black corresponds to decrease inEgfrtranscription levels). Other genes may also be involved in generating quantitative size variation (dashed black lines). The level ofEgfrtranscription then translates to quantitative size variation of worker larvae (solid black lines). Finally, we infer that the continuous size distribution of final size worker larvae translates into the continuous size distribution of adult workers (dashed black lines). Figure 5: Model for the generation of a continuous distribution of worker size through quantitative DNA methylation of Egfr . Solid black lines indicate our results, whereas dashed black lines indicate our inferences from the literature. Lines with perpendicular tips indicate repression, whereas lines with arrowheads indicate activation. Environmental variation may lead to either global DNA hyper- or hypo-methylation (dashed black lines). Intermediary genes or processes quantitatively modulate this global DNA methylation state (solid black lines) into a specific level of Egfr methylation (black lollipops and box with increasing gradient from left to right, where an increase in black corresponds to increasing levels of methylation), which results in a specific level of Egfr transcription level (box with decreasing gradient from left to right, where a decrease in black corresponds to decrease in Egfr transcription levels). Other genes may also be involved in generating quantitative size variation (dashed black lines). The level of Egfr transcription then translates to quantitative size variation of worker larvae (solid black lines). Finally, we infer that the continuous size distribution of final size worker larvae translates into the continuous size distribution of adult workers (dashed black lines). Full size image In ants, Egfr may be positioned as a key regulator of conserved pathways; in honeybees, diet activates EGFR to regulate several important downstream pathways, including the TOR, juvenile hormone and insulin signalling pathways [39] . In other animals, EGFR signalling is also known to play a role in regulating DNA methylation through downstream activation of DNMTs [49] resulting in altered cellular growth. This raises the possibility that in ants, Egfr may not only be a target of DNA methylation but may in turn also regulate DNA methylation. It is important to note that the main goal of our study was to understand the developmental role of DNA methylation in producing quantitative variation in worker size and not caste determination, that is, producing minor and major worker subcastes with their discrete allometric differences between head and body size ( Fig. 1c ). Caste determination is a complex process that may require more than just a size increase through Egfr . Major worker subcastes have many discrete features other than size [11] , which are not present in minor worker subcastes, and may require juvenile hormone and other factors. The quantitative methylation of specific loci, like Egfr , may represent a more general mechanism for the generation and evolution of quantitative trait variation across animals. DNA methylation, the EGFR pathway and specific pathways downstream of EGFR are highly conserved across animals, and DNA methylation is known to be transgenerationally inherited [9] , [50] , [51] , [52] . In vertebrates, quantitative differences in methylation of an inserted retroviral element in front of the Agouti gene in mouse defines differences in coat colour [53] , and the distribution of coat colours could be shifted by altering the methyl content in maternal diet [53] . It remains to be shown, however, whether natural inter-individual epigenetic variation of this inserted retroviral element generates variation in coat colour in natural populations. This mechanism may also underlie associations found between epigenetic variation and disease susceptibility, like that found for Type II diabetes in humans [54] , as well as quantitative traits, like that found for flowering time and height in plants [51] . Finally, our results hold important implications for quantitative genetics. The eventual unification of Mendelian inheritance with Darwin’s theory of natural selection was made possible by the infinitesimal model [55] , which assumes that quantitative trait variation is generated by the action of an infinite number of loci that have small and equal effects on the phenotype [3] , [56] . The evolution of quantitative traits is therefore thought to occur through random mutations across these loci [3] , [56] . However, the empirical search for QTLs has revealed that trait variation often maps to specific genetic regions of small or large effect, and with specific functions [4] , [57] . The apparent gap between the assumptions of the infinitesimal model and the results of QTL analyses is further exacerbated by the fact that countless studies have demonstrated that QTLs cannot in themselves explain all heritable variation underlying quantitative traits [5] , such as growth or size in humans [58] , Arabidopsis [59] and yeast [60] . These difficulties underscore the many challenges that remain in understanding the genetic basis of quantitative trait variation [3] , [5] . Our findings may help resolve these outstanding challenges in the field of quantitative genetics because they show that the phenotypic possibilities of a genetic locus may be determined by both genetic variation and the influence of the environment through quantitative DNA methylation. Therefore, alongside genetic variation, the environment can generate a vast array of quantitative trait variation in natural populations. Collection of samples We collected mated queens from Tallahassee, Florida, USA. Mature colonies originating from single queens were maintained in plastic boxes with glass test tubes filled with water constrained by cotton wool, and were fed a combination of mealworms, crickets, fruit flies and Bhatkar-Whitcomb diet as in Rajakumar et al . [16] All colonies were maintained at 27 °C, 70% humidity and 12 h day:night cycle. Larval and adult sampling, genotyping and pharmacological experiments were conducted on a single colony to control for colony and population variation and began after the colony had matured for approximately 4 years. In order to conduct SAM (luminometric methylation assay (LUMA)), 5-AZA-dC (LUMA) and EGFRi (western blot) validation assays, which are described in more detail below, we pooled samples to be treated from multiple colonies because the assays required a significant amount of material. Determination of the number of instars for worker larvae To describe the epigenetic status of specific developmental stages of larval development, the number of larval instars was determined. The colony which larvae were taken from was not in the process of producing reproductives (males or queens). This is important because larvae of Camponotus species that become reproductive have been suggested to have a different number of instars compared with worker larvae [61] . To discriminate between instars, widths of the head capsules of larvae were measured as previously described [62] . Larvae analysed that were designated as minor ‘m’ or major ‘M’ worker larvae are terminal larvae, meaning that they have reached the end of larval development, which we have determined is at the end of the fourth instar. m and M worker larvae share the same head capsule size but differ in overall body size. A larvae is classified as terminal if it meets the two following requirements: the gut of the larvae is completely black and the fat cells of the larvae are at peak density and completely engulf the gut [63] . When the larvae exhibit those two characters, then they are at their terminal stage. Larvae designated m or M that were used specifically for analysis (LUMA, bisulfite sequencing, quantitative-PCR) were the smallest and largest terminal larvae, respectively, in order to ensure their fate. Adults described as m or M is designated as such based on allometric differences (detailed in ‘Measuring of adult workers’ section). Culturing of pharmacologically treated larvae To determine the role of methylation during worker larval development, early 4th instar (the last instar based on Fig. 1d ) larvae were selected for methylome and EGFR signalling manipulation. SAM, a methyl donor to DNA methyltransferases [38] (B9003S, New England Biolabs), was applied at a concentration of 32 mM (dissolved in 10% ethanol and 0.005 M sulfuric acid). 5-AZA-dC, a cytidine analogue inhibitor of DNA methylation [37] (A3656, Sigma-Aldrich), was applied at a concentration of 10 mM (dissolved in water). Last, the highly specific and potent quinazolone EGFR inhibitor, PD153035, which acts through the suppression of epidermal growth factor-dependent EGFR phosphorylation [44] (234491, EMD Millipore), was applied at a concentration of 10 μM (dissolved in dimethylsulphoxide). Larvae were isolated and placed laterally on a Petri dish with the aid of a microscope. A volume of 4 μl of solution was then applied topically allowing for absorption and larval feeding. After treatment, larvae were setup in plastic boxes and fed in the same manner as colonies. For each treatment, 40 larvae were treated and 80 adult minor workers were supplemented to the box to care for them. Half of the larvae were collected at the end of larval development for further quantitative gene expression as well as pyrosequencing, while the other half were left to develop. Timing of eclosion (the beginning of adulthood) was monitored for the remaining larvae of each treatment. Newly emerged adults were subsequently measured to detect any morphological effects of the drug treatments. To validate effects of SAM and 5-AZA-dC on global methylation levels, 50 larvae treated with SAM, 5-AZA-dC and their respective controls were collected for LUMA. Measuring of adult workers Workers were measured for several parameters for the purpose of identifying any shifts in size that might have been caused by the manipulation of larval methylation or EGFR signalling inhibition. In particular, we measured scape length, head width, thorax length, thorax width and mandible length as in Diniz-Filho (1994). In Camponotus , Diniz-Filho (1994) found that head width exhibited positive allometry ( Fig. 1c ), whereas scape length was isometric and suggested that for a bivariate analysis of allometry, scape length could be used as an independent variable (due to its isometry) [64] . Isometric measures, like scape length, are highly correlated and proportional to body size [64] and therefore serve as independent and accurate proxies for body size to examine the size frequency of individuals of a colony. In a similar manner, head width and scape length were used in another Camponotus species [65] as well as other polymorphic ant species [11] . An added advantage for measuring the length of the scape is its simplicity and therefore it reduces any technical variation in measurements between individuals. Therefore, to determine the relative distribution of sizes ( Fig. 1a,b ), we used scape length as a proxy for body size. By characterizing the allometry found within the continuous size distribution of workers, we could classify minor (m) and major (M) worker adults ( Fig. 1a,c ). Microscopy We used a Zeiss Discovery V12 stereomicroscope and Zeiss Axiovision software to measure the larvae (in μm) and adults (in μm). For larval imaging, we used an Olympus TM3000 tabletop scanning electron microscope. DNA and RNA extraction Larvae were collected and pooled ( n =20) for each instar and immediately frozen at −80 °C. Since our trait of interest, size, is a variable specific to a large proportion of cells within the animal, we assumed that heterogeneous tissues across individual larvae would still provide data relevant to size as a trait. DNA and RNA were both extracted using Allprep DNA/RNA extraction kits (80204, Qiagen) as instructed for animal tissues. Homogenization of samples was achieved using RLT+ provided with pestle grinding. Individual larvae selected at the fourth instar were also processed in a similar manner. A DNAse on-column step was done in all samples during RNA extraction. All samples were quantified using Nanodrop 1000 (Thermo Scientific). Luminometric methylation assay LUMA is a high-throughput assay used to determine global (genome-wide) DNA methylation. The LUMA method used in our study is a modification described by Karimi et al . [66] LUMA involves the digestion of genomic DNA by a methylation-sensitive ( HPA II) or -insensitive ( MSPI ) restriction enzymes in combination with an internal control restriction enzyme ( Eco RI) to normalize the DNA input. Eco RI (FD0274), Hpa II (FD0514) and Msp I (FD0541) were all purchased from Thermo Scientific. Both Hpa II and Msp I restriction enzymes recognize and cleave 5′-CCGG-3′ sequences producing 5′-CG overhangs, whereas Eco RI recognizes and cleaves 5′-GAATTC-3′ sequences and produces 5′-AATT overhangs. The extent of cleavage is determined by a bioluminetric polymerase extension assay, which measures the filling in of the sticky ends generated by the enzymatic digestion using a four-step pyrosequencing reaction. Samples were incubated (37 °C, 4 h) and then heat inactivated (80 °C, 20 min). Digested genomic DNA (15 μl) was mixed with pyrosequencing annealing buffer (15 μl; Qiagen). Samples were transferred to 24-well pyrosequencing plates for sequencing (PyroMark 24; Biotage). Peak heights for C and A represent the Hpa II and Msp I cuts (methylation) and Eco RI (input DNA), respectively. The formula to calculate an index of genomic methylation is: [MspI (C)/ EcoRI (A)]/[HpaII (C)/ EcoRI (A)]. The higher the ratio between Msp I cuts (cleaves all CCGG sites) and Hpa II cuts (cleaves only unmethylated CCGG), the higher the methylation level. All samples were run in triplicate. This method only measures an absolute index of methylation across the entire genome so equal bidirectional differences in DNA methylation are unlikely to register observable differences. Bisulfite mapping, sequencing and expression analyses DNA was treated with sodium bisulfite and primers ( Supplementary Table 1 ) were designed for converted products of the 5′ region (based on Kamakura, 2011) of C. floridanus Egfr (scaffold 550: bp113394-bp113619; located using GBrowse of the Hymenoptera Genome Database [67] Bankit ID KP325210). Bisulfite conversion was done with Epitect Bisulfite Conversion kit (Qiagen). Bisulfite PCRs were amplified using two rounds of PCR using outer and nested primers (see Supplementary Table 1 ). Cycling conditions involved an initial step of 5 min at 95 °C followed by 35 cycles of 95 °C for 1 min, T m for 2.5 min, 72 °C for 1 min and followed by 5 min of 72 °C. PCR products were sequenced using the Biotage Pyrosequencer as previously described [68] . For all samples, 500 ng of RNA was subjected to RT–PCR according to manufacturer’s protocols (Roche) and quantified using quantitative PCR on the Lightcycler 480 (Roche). Primers for all genes ( Supplementary Table 1 ) were created across exon boundaries. As a housekeeping gene, we used RPS49 for normalization as it was previously shown to have stable expression both across larval development and following juvenile hormone manipulation in Apis mellifera [69] . Quantitative PCR was amplified with a pre-incubation at 95 °C for 10 min followed by 45 cycles of 95 °C for 10 s, 60 °C for 10 s, 72 °C for 10 s followed by 10 min of 72 °C. In vitro luciferase assay The 5′ region of Egfr corresponding to that described in A. mellifera [39] was amplified using the ‘Luciferase construct PCR primers’ ( Supplementary Table 1 ) generating a 378-bp fragment of the 5′ region of the C. floridanus Egfr gene (scaffold 550: bp113394-bp113772; located using GBrowse of the Hymenoptera Genome Database [67] ). Bam HI and Hin dIII restriction sites were incorporated into the primers in order to generate restriction sites to clone the fragment into the CpG-less pCpGl (ref. 70 ) in 5′ to 3′ (sense) or 3′ to 5′ (antisense) orientation, respectively. As the vector does not contain CpG sites, all methylated sites are contained in the Egfr 5′ region. The constructs were methylated in vitro with SssI CpG DNA methyltransferases (M0226L, New England Biolabs) as previously described [68] . Transfections were performed using calcium phosphate precipitation as described previously into HEK293 cells (CRL-1573, American Type Culture Collection). Cells were harvested 48 h after transfection and luciferase activity was assayed using the Luciferase Assay System (Promega). Western blotting analyses Fifty larvae treated with dimethylsulphoxide or EGFR inhibitor were collected 24 h after treatment and homogenized in RIPA buffer (1 × PBS, 1% NP-40, 0.5% sodium deoxycholate, 0.1% SDS and 1 × complete protease inhibitors; Roche Diagnostics). Total protein yield was determined using Bradford assay (Bio-Rad) and a total of 30 μg of protein was loaded onto a 10% SDS–polyacrylamide gel electrophoresis. As adapted from bees [39] , protein extracts were immunoblotted with anti-EGFR (sc-33746, Santa Cruz Biotech) and anti-phosphotyrosine PY20 antibody (525295, Millipore) at 1:1,000 dilution. EGFR was then blotted by a secondary anti-rabbit (sc-2004, Santa Cruz Biotech) and PY20 was blotted by anti-mouse at 1:5,000 dilution. For quantification, total EGFR was determined with anti-EGFR followed by stripping at pH 6.8 and re-blotting with anti-phosphotyrosine in triplicates to determine overall tyrosine posphorylation. The intensities of the signals were then quantified using Image J software and total phosphorylation was measured and presented as the ratio between the intensity of the phosphorylated band corresponding to EGFR divided by intensity of total EGFR. EGFR genotyping in adults Minor ( n =9) and major ( n =8) representing the extremes of adult development (a and e, see Fig. 1B ). Abdomens were removed from adults to exclude exogenous DNA from gastrointestinal microbiota. Template DNA was used with primers used to amplify the EGFR locus used for luciferase promoter constructs (see Supplementary Table 1 ). Cycling conditions involved an initial step of 5 min at 95 °C followed by 35 cycles of 95 °C for 1 min, 60 °C for 2.5 min, 72 °C 1 min, followed by 5 min of 72 °C. PCR products were performed at the Génome Québec Innovation Centre (Montréal, Canada) using both forward and reverse primers. Statistical analysis All data are expressed as mean±s.e.m., except developmental time, which is expressed as standard deviation (s.d.) and morphometrics in the form of box-and-whisker plots. Comparisons between groups were performed using two-tailed, unpaired Student’s t -test, except in the case of unequal variance for which the Mann–Whitney U -test was performed. Multivariate analysis of variance performed considered all morphometric traits, significance was set at P <0.05 and Pillai’s Trace was used. Correlations of percent methylation with terminal larval size were calculated using Pearson correlation and significance was initially set at P <0.05 followed by Bonferroni correction for multiple tests, implemented to correct for multiple comparisons. Statistical analysis was undertaken using Prism (GraphPad Software Inc.) except for multivariate analysis of variance, which was performed in R. Accession codes. The Egfr promoter sequence generated in this study has been deposited in NCBI nucleotide database under accession code KP325210. How to cite this article: Alvarado, S. et al . Epigenetic variation in the Egfr gene generates quantitative variation in a complex trait in ants. Nat. Commun. 6:6513 doi: 10.1038/ncomms7513 (2015).